Evidence for photogenerated intermediate hole polarons in ZnO Despite their pronounced importance for oxide-based photochemistry, optoelectronics and photovoltaics, only fairly little is known about the polaron lifetimes and binding energies. Polarons represent a crucial intermediate step populated immediately after dissociation of the excitons formed in the primary photoabsorption process. Here we present a novel approach to studying photoexcited polarons in an important photoactive oxide, ZnO, using infrared (IR) reflection–absorption spectroscopy (IRRAS) with a time resolution of 100 ms. For well-defined (10-10) oriented ZnO single-crystal substrates, we observe intense IR absorption bands at around 200 meV exhibiting a pronounced temperature dependence. On the basis of first-principles-based electronic structure calculations, we assign these features to hole polarons of intermediate coupling strength. Although polarons are crucial for optoelectronics, photovoltaics and photochemistry [1] , little is known about polaron lifetimes and binding energies (BEs) [2] , [3] , [4] . More information on polaronic states is urgently needed, particularly for enhancing our understanding of photochemistry, where the most promising results are expected to come from well-defined, monocrystalline system, for example, ZnO(10-10) substrates. The photophysics of oxides consists of a cascade of processes. A decay of the short-lived (ps timescale) excitons created in the initial photoabsorption process leads to polaron formation. For ZnO, a wide-bandgap metal oxide with desirable physical and chemical properties, only indirect experimental [2] and limited theoretical [4] , [5] information on the existence of polarons is available: theoretical description of large (weak coupling) electron polarons agrees with experimental observation [2] , [5] ; and small (strong coupling) polarons are not stable [6] . This contrasts with excitons, which have been studied in detail and whose lifetimes (around 60 ps (ref. 7 )) and BEs (60 meV (refs 8 , 9 )) have been determined. After the dissociation of the photoinduced exciton, the charge carriers—free electrons and free holes—may be trapped in polaronic states, which in turn can diffuse through the crystal. When the carriers reach the surface, they can trigger reactions in the adsorbed chemical species [1] , [10] , [11] , [12] . Compared with the ultrafast formation dynamics of excitons in ZnO(10-10) single crystals [7] , polaron formation involves the motion of nuclei and thus occurs on a much longer timescale. In the following, we present a novel approach to studying the photoexcited polarons in zinc oxide (ZnO) using infrared (IR) reflection–absorption spectroscopy with a time resolution of 100 ms employing the so-called rapid scan method, where interferograms are acquired in rapid succession with the mirror moving at the highest possible speeds. The time resolution is the time needed to record a single interferogram, in this case 100 ms. In well-defined (10-10) oriented ZnO single crystals, we observe pronounced absorption bands at around 200 meV in IR spectra under ultra-high vacuum conditions—a sharp feature and an absorption edge (AE)-like feature. These previously unobserved strong bands exhibit a temperature-dependent lifetime, and through first-principles-based electronic structure theory calculations [4] , [6] , [13] , [14] , [15] , we attribute them to a hole polaron of intermediate coupling strength. Taken together, the ground-breaking observation and attribution of intermediate polarons will trigger a new era of polaron research. Ultraviolet-induced features in time-resolved IRRAS data We created polarons by ultraviolet illumination and probed their behaviour with IR absorption. In the difference IR spectra shown in Fig. 1a , recorded after illuminating (365 nm, 8 W) the sample (see experimental methods) for 10 min at 118 K, we identify several well-defined ultraviolet-induced features: a single, sharp peak at 1,288 cm −1 (160 meV), most prominent for p-polarized light, and an AE-like feature with an apparent AE at around 1,630 cm −1 (202 meV) superimposed with a fine structure peaked at 1,790 and 2,140 cm −1 . After switching off the ultraviolet illumination, the intensity of these ultraviolet-induced features quickly decreased (see Fig. 1c ). The lifetime, that is, the time constant of the decaying signal, was 25 s at 75 K and dropped to 14 s at 140 K (data not shown). We were also able to follow the ultraviolet-induced appearance of these features, see Fig. 1b (see, for example, Supplementary Fig. 1 ). 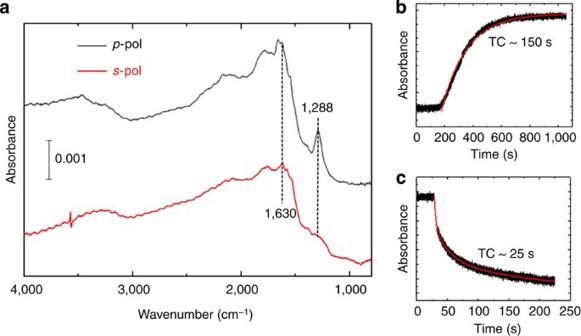Figure 1: Steady state (during ultraviolet light irradiation) IR spectra. Steady state (during ultraviolet light irradiation) IR spectra (p- ands-polarization) of ZnO(10-10) recorded at 118 K (a). Time dependence of the intensity of the sharp feature at 1,630 cm−1on starting (b) and terminating (c) ultraviolet irradiation at 75 K with the time constants (TC) indicated for the rise and decay of the signal. The corresponding rapid scan IR spectra are shown in theSupplementary Fig. 1. Figure 1: Steady state (during ultraviolet light irradiation) IR spectra. Steady state (during ultraviolet light irradiation) IR spectra ( p - and s -polarization) of ZnO(10-10) recorded at 118 K ( a ). Time dependence of the intensity of the sharp feature at 1,630 cm −1 on starting ( b ) and terminating ( c ) ultraviolet irradiation at 75 K with the time constants (TC) indicated for the rise and decay of the signal. The corresponding rapid scan IR spectra are shown in the Supplementary Fig. 1 . Full size image The intensity of the ultraviolet-induced IR features after saturation is strongly temperature dependent, see Fig. 2 . An Arrhenius analysis of the intensity of the sharp feature at 1,630 cm −1 as a function of substrate temperature yields an (apparent) activation energy of 245 meV. Attempts to observe these ultraviolet-induced features in IR spectra recorded in transmission geometry for ZnO powders (analogous to r-TiO 2 (ref. 16 )) were unsuccessful due to the enormous IR absorption caused by the excitation of bulk optical phonons (see ZnO crystal data, Supplementary Fig. 2 and Supplementary Note 1 ). 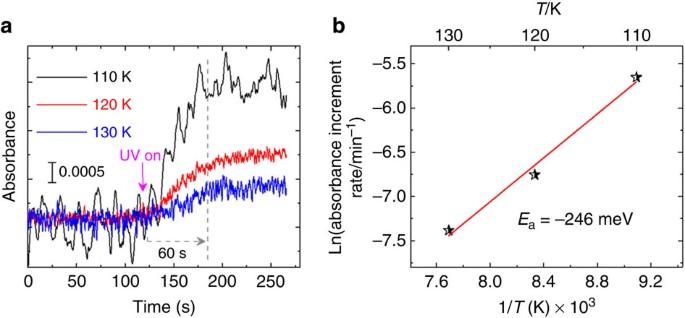Figure 2: The transients of IR absorbance. The transients of IR absorbance rises from a ZnO(10-10) single crystal after initiation of the ultraviolet light excitation at 110, 120 and 130 K (a) and corresponding Arrhenius plot of the initial rates of IR absorbance increase and sample temperatures (b). Figure 2: The transients of IR absorbance. The transients of IR absorbance rises from a ZnO(10-10) single crystal after initiation of the ultraviolet light excitation at 110, 120 and 130 K ( a ) and corresponding Arrhenius plot of the initial rates of IR absorbance increase and sample temperatures ( b ). Full size image The ultraviolet-induced features in the IR absorption spectra of ZnO we observed after exposure to ultraviolet light have not—to our knowledge—yet been reported. Since the excitons generated in the photoabsorption process have lifetimes of less than 60 ps (ref. 17 ), they cannot account for these new bands. We thus assign the ultraviolet-induced features to polaronic states, analogous to the case of TiO 2 (ref. 16 ). If the excitations we observed for ZnO were due to electron polarons, chemical and photon electron doping should yield similar results. This was indeed the case for r-TiO 2 , where IR spectra recorded after exposure to atomic H (chemical doping, leading to an n -doping of TiO 2 ) were very similar to those recorded after ultraviolet exposure (photon doping) [16] . Since spectra recorded after n -doping resulting from exposure to D-atoms [18] , [19] , [20] (see Supplementary Fig. 3 ) are clearly different from those recorded after ultraviolet exposure, we therefore regard the effects observed in the IR spectra as evidence for hole polarons. Accordingly, we assign the broad feature starting at 1,630 cm −1 , which is reminiscent of an AE, to a transition of electrons from the top of the valence band (VB) into a hole polaronic state. The fine structure superimposed on the AE is attributed to different densities of states of electronic states deeper in the VB. The sharp feature visible at 1,288 cm −1 in our data must have a different physical character. First, this peak shows pronounced polarization dependence, while the fine structure of the AE feature is only mildly affected (see Fig. 1a ). Second, longer exposures to ultraviolet light at 73 K showed saturation effects for the AE feature but not for the 1,288 cm −1 peak. Theoretical analysis of polarons in ZnO To interpret experimental observations, we carried out a thorough theoretical analysis. We distinguish between large and small electron and hole polarons. Large ones are trapped by strong self-induced lattice distortions, and small polarons correspond to an electron in the bottom of the conduction or a hole in the top of the VB. The electron or hole energy is renormalized by the electron–phonon interaction. Polaron BEs were calculated from first principles using the Fritz Haber Institute ab initio molecular simulations (FHI-aims) code [21] and the Heyd–Scuseria–Ernzerhof hybrid density-functional (HSE06) [6] , [13] , see computational methods. The computed BEs are 33 meV for the large electron and 81 meV for the large hole polaron. Neither small electron nor small hole polarons are stable in ZnO, in agreement with the results of Varley et al . [4] , also not at larger fractions of exact exchange in the HSE functional. Currently, no first-principles theory is available to describe the optical absorption spectrum of polarons. We therefore resort to the commonly-applied Fröhlich model (see refs 22 , 23 ) in which the strength of the electron–phonon coupling is determined by the effective mass m * of the charge carrier: Here ω LO is the longitudinal optical (LO) phonon frequency, and ɛ ∞ and ɛ 0 are the electronic and ionic dielectric constants, respectively. We have previously calculated the effective masses of the band edges [15] . The conduction edge features one band with m c =0.24 m e (where m e is the free electron mass) that originates from Zn s-orbitals. The highest VBs are mainly of O 2p-character. Because wurtzite has no cubic symmetry, unlike zinc-blende, the top of the VB is not threefold degenerate and the effective masses perpendicular ( m perp =0.4 m e ) and parallel ( m par =2.7 m e ) to the c axis differ. The corresponding coupling strengths are α c =0.95, α perp =1.2 and α par =3.1. We have cross-checked the analytic Fröhlich model for the coupling strength of LO modes with density-functional perturbation theory calculations for GaN and found them to be in excellent agreement [14] . We expect the same for ZnO. According to common polaron classification schemes [22] , [23] , α ∼ 1 or lower corresponds to a large polaron, α >5 is indicative of a small polaron and values in between have intermediate coupling strength. In ZnO, we should therefore have one large electron, one large hole polaron and an additional intermediate hole polaron. Such intermediate polarons cannot currently be treated with first principles theories. Using Feynman’s path integral expansion for the polaron BE in terms of α (ref. 22 ) we obtain E c =70 meV, E perp =90 meV and E par =240 meV. E c and E perp are of the same order as our HSE06 results for the large polarons. E par , however, is larger and in remarkably good agreement with the experimental activation energy of 245 meV. For large and intermediate polarons, the onset of absorption in the IR spectrum does not correspond to the polaron BE. Numerical results for the optical absorption spectrum of the Fröhlich model [24] , [25] reveal that the peak maximum in the IR spectrum shifts from just above the LO frequency at α =1 to about 2.5 · ω LO for α =3.1. With LO frequencies of 577 cm −1 and 590 cm −1 in ZnO [2] , we obtain for the intermediate hole polaron a peak maximum at ∼ 1,500 cm −1 , in remarkably good agreement with the AE position in the experimental data. HSE06 band structure calculations for the ZnO (10-10) surface yield hole masses of 0.41 m e perpendicular and 2.02 m e parallel to the c axis of the ZnO bulk. The corresponding α par =2.8 at the surface is thus slightly smaller than in the bulk, and the associated polaron peak moves to lower energies. We attribute the polarization-dependent feature at 1,288 cm −1 in the experimental spectra to an intermediate surface polaron. The theoretical peak positions are consistent with the spectrum shown in Fig. 1 , which confirms our assignment of the experimental features as hole polarons of intermediate coupling strength. Note that the AE features of the large electron and hole polarons with a coupling parameter α of 1 are expected to lie in the region of the LO frequencies, that is, around 600 cm −1 . As this frequency is below the cutoff of our IR detector, these features cannot be seen in our experiments. Our data demonstrate that IR spectroscopy, using reflection geometry in connection with single-crystal surfaces, is well suited to probe ultraviolet-induced polarons in ZnO. On the basis of our theoretical analysis, we assign the AE-like feature at around 202 meV to hole polarons of intermediate coupling strength. The experimental findings reported here have important implications for the photochemical properties of ZnO. Our results confirm the absence of small electron polarons in ZnO—in agreement with chemical intuition—but strongly suggest the presence of hole polarons of intermediate coupling strength. Such pseudoparticles have not yet been considered in the photophysics and photochemistry of ZnO. Regarding the latter, for hole-accepting molecular species, the hole polaron BE reported here has to be considered for understanding the details of the photocatalytic process. Clearly, the present findings call for more extensive experimental and theoretical studies of polarons in ZnO and other oxides. In particular, our analysis points to two deficiencies in the theoretical state of the art; we need a first-principles theory for polarons at intermediate coupling strengths, and the optical absorption spectrum of polarons. Experimental methods The samples (CrysTec, Germany; size 10 × 10 mm) were mounted in an ultra-high vacuum chamber (base pressure <2 × 10 −10 mbar) equipped with devices to allow for a thorough complementary sample characterization using X-ray photoelectron spectroscopy and low-energy electron diffraction. The sample surface was cleaned using standard procedures [2] including Ar+ ion sputtering and annealing steps until the sample was clean (as judged from X-ray photoelectron spectroscopy data) and well-ordered (as judged from the presence of well-defined spots in the low-energy electron diffraction pattern). IR reflection–absorption spectra were recorded with a commercial instrument (Bruker Vertex 80v) and normalized by subtraction of a reference spectrum recorded before illumination. Computational methods To compute the self-trapping energy of small electron or hole polarons, an additional electron or hole was added to a 96-atom supercell of ZnO using the method described in refs 1 , 4 ), and the atomic structure was fully relaxed in HSE06. To compute the BEs of large electron or hole polarons, we evaluated the second derivatives of the HSE06 eigenvalues associated to the bottom of the conduction and the top of the VB with respect to the phonon displacements following Antonius et al . [6] We used a 6 × 6 × 8 electronic k-point and a 6 × 6 × 4 phonon q-point mesh. Polaron BEs are referenced to the band edge positions before renormalization. How to cite this article: Sezen, H. et al . Evidence for photogenerated intermediate hole polarons in ZnO. Nat. Commun. 6:6901 doi: 10.1038/ncomms7901 (2015).